Live imaging of calcium spikes during double fertilization inArabidopsis Ca 2+ waves and oscillation are key signalling elements during the fertilization process of animals, and are involved, for example, in egg activation. In the unique double fertilization process in flowering plants, both the egg cell and the neighbouring central cell fuse with a sperm cell each. Here we succeeded in imaging cytosolic Ca 2+ in these two cells, and in the two synergid cells that accompany the gametes during semi- in vivo double fertilization. Following pollen tube discharge and plasmogamy, the egg and central cells displayed transient Ca 2+ spikes, but not oscillations. Only the events in the egg cell correlated with the plasmogamy. In contrast, the synergid cells displayed Ca 2+ oscillations on pollen tube arrival. The two synergid cells showed distinct Ca 2+ dynamics depending on their respective roles in tube reception. These Ca 2+ dynamics in the female gametophyte seem to represent highly specific signatures that coordinate successful double fertilization in the flowering plants. Ca 2+ is important as an intracellular second messenger in the fertilization of many organisms [1] , [2] , [3] . In animals including mouse, xenopus, ascidian, starfish and sea urchin, various patterns of cytosolic Ca 2+ waves and oscillations are involved in fertilization and the subsequent onset of embryogenesis [3] , [4] . In flowering plants, the egg is intimately associated with typically six to eight other haploid cells forming the female gametophyte. These include the central cell representing the second female gamete and two synergid cells that produce the signals, which guide the male gametophyte, or pollen tube, towards the ovule. The pollen tube delivers two non-motile sperm cells whose release occurs by bursting, which in turn is triggered when the tube interacts with the synergid cells [5] . The receptive synergid cell degenerates following this interaction, whereas the other synergid cell persists. After their ejection from the pollen tube, the two sperm cells stay immobile between the two female gametes for several minutes and subsequently fuse with the egg and central cells, respectively [6] . These two fusion events give rise to the embryo and to the endosperm, respectively, and the process is therefore termed double fertilization. Since the entire fertilization process takes place within the ovule, characterization of Ca 2+ dynamics in the egg cell in situ and in the accompanying gametophytic cells has been elusive in plants. Previously, in vitro fertilization of isolated egg cells [7] , [8] , [9] has shown Ca 2+ influx in the vicinity of the sperm entry site and waves of Ca 2+ influx were observed to spread through the whole egg cell plasma membrane [10] , [11] . This Ca 2+ influx may trigger egg activation, which includes cell wall formation and vacuole fragmentation [12] . The coordination of this process in vivo is likely to require intimate cell-to-cell communication between the gametophytic cells [13] . Assessing the complete picture of the signalling processes therefore requires the presence of the other gametophytic cells. Although Ca 2+ imaging has been performed to monitor the interaction between the synergid cell and the pollen tube [14] , Ca 2+ dynamics during the actual gamete fusion is unknown. Here, we show Ca 2+ dynamics of the female gametophytic cells in semi -in vivo condition by using the Ca 2+ probe Yellow Cameleon 3.60 (YC3.60) (ref. 15 ) and high-resolution microscopies. The egg cell revealed two Ca 2+ spikes following pollen tube discharge and plasmogamy. The central cell displayed similar Ca 2+ spikes with the first one occurring on pollen tube discharge but the second spike not always being correlated with the plasmogamy. The two synergid cells on the other hand displayed very different Ca 2+ dynamics. Both synergid cells showed Ca 2+ oscillations on pollen tube arrival. Ca 2+ was higher in the receptive synergid, but oscillations were sustained in the persistent synergid after double fertilization. The data suggest that characteristic Ca 2+ signalling in the principal female gametophytic cells is involved in successful double fertilization in plants. Two Ca 2+ spikes in the egg cell during double fertilization To monitor cytosolic Ca 2+ dynamics in the egg cell of Arabidopsis thaliana , the Ca 2+ probe Yellow Cameleon 3.60 (YC3.60) (ref. 15 ) was expressed under the egg cell-specific promoter DD45 (ref. 16 ). Ovules expressing this YC3.60 sensor were cultivated with pollen tubes for semi- in vivo double fertilization [6] , [17] . In this setup, the female gametophyte is intact and still surrounded by the ovule tissues. To visualize behaviour of sperm cells, their nuclei were labelled with the red fluorescent protein mRFP fused to the histone H3.3 variant HTR10 (ref. 6 ). We at first performed two-photon excitation imaging, which enabled us to simultaneously excite CFP and mRFP without any time lag using the 800 nm excitation wavelength [18] and to obtain high-resolution imaging within the depths of the ovule [6] . On the basis of the movement of sperm cell nuclei, the timing of pollen tube discharge, egg cell fertilization and central cell fertilization were evaluated as previously reported [6] . The rapid movement of the sperm cell nuclei is indicative of pollen tube discharge. After a short period of immobility, the sperm cell nuclei resume movement towards the target female gamete cells representing fertilization (plasmogamy) [6] , [19] . We observed two transient peaks of the cytosolic Ca 2+ concentration ([Ca 2+ ]cyt) in the egg ( Fig. 1b,c , Supplementary Movie 1 , Supplementary Fig. 1a ), which appeared correlated in time with pollen tube discharge and egg cell fertilization, respectively. There was no clear Ca 2+ change detected in the egg at the timing of central cell fertilization ( Fig. 1b,c ). 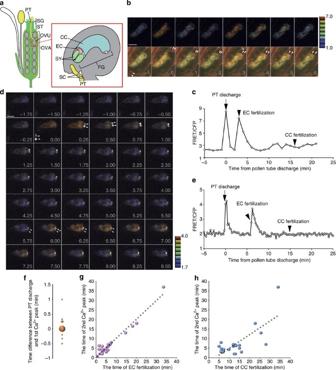Figure 1: Two Ca2+spikes detected in the egg cell during double fertilization. (a) Scheme of fertilization process in flowering plants. A pollen grain containing the two sperm cells (SC) adheres to the stigma (SG), then produces a pollen tube (PT), which enters the style (ST) and grows towards the ovary (OVA). Finally, the pollen tube arrives at the ovule (OVU). After the pollen tube reaches the female gametophyte (FG), one of the synergid cells (SY) degenerates and the pollen tube bursts to discharge its contents into the female gametophyte. One sperm cell fuses with the egg cell (EC) to form the embryo, and the other fuses with the central cell (CC) producing the endosperm. (b) Time-lapse series of two-photon excitation YC3.60 images (maximum projection of three optical sections) of the egg cell before and after pollen tube discharge. Upper panels show representative FRET/CFP ratio images. Lower panels show merged images of CFP (cyan), Venus (yellow) and mRFP (red), which labels sperm cell nuclei with pHTR10::HTR10-mRFP. Arrowheads indicate sperm cell nuclei. Asterisk shows the timing of egg cell fertilization. Numbers indicate time (min); the frame showing rapid movement of sperm cells was designated the onset of the pollen tube discharge, that is, time 0. Scale bar, 10 μm. (c) Time course of the FRET/CFP ratio change shown inb. (d) Time-lapse series of confocal optical sections (single optical sections) of the egg cell expressing YC3.60 before and after the pollen tube discharge. Sperm cell nuclei were labelled with pRPS5A::H2B-tdTomato (white in colour). Arrowheads emphasize the movement of sperm cell nuclei just before and after pollen discharge and egg cell fertilization. Asterisk shows the timing of egg cell fertilization. Scale bar, 10 μm. Numbers indicate time (min) as inb. (e) Time course of the FRET/CFP ratio change shown ind. (f) Plot of the time difference between pollen tube discharge and first Ca2+peak (n=28). (g,h) Plot of the timing of events relating the second Ca2+peak with EC fertilization (g,n=24) or CC fertilization (h,n=21). A regression line (dashed line) is shown. Figure 1: Two Ca 2+ spikes detected in the egg cell during double fertilization. ( a ) Scheme of fertilization process in flowering plants. A pollen grain containing the two sperm cells (SC) adheres to the stigma (SG), then produces a pollen tube (PT), which enters the style (ST) and grows towards the ovary (OVA). Finally, the pollen tube arrives at the ovule (OVU). After the pollen tube reaches the female gametophyte (FG), one of the synergid cells (SY) degenerates and the pollen tube bursts to discharge its contents into the female gametophyte. One sperm cell fuses with the egg cell (EC) to form the embryo, and the other fuses with the central cell (CC) producing the endosperm. ( b ) Time-lapse series of two-photon excitation YC3.60 images (maximum projection of three optical sections) of the egg cell before and after pollen tube discharge. Upper panels show representative FRET/CFP ratio images. Lower panels show merged images of CFP (cyan), Venus (yellow) and mRFP (red), which labels sperm cell nuclei with pHTR10::HTR10-mRFP. Arrowheads indicate sperm cell nuclei. Asterisk shows the timing of egg cell fertilization. Numbers indicate time (min); the frame showing rapid movement of sperm cells was designated the onset of the pollen tube discharge, that is, time 0. Scale bar, 10 μm. ( c ) Time course of the FRET/CFP ratio change shown in b . ( d ) Time-lapse series of confocal optical sections (single optical sections) of the egg cell expressing YC3.60 before and after the pollen tube discharge. Sperm cell nuclei were labelled with pRPS5A::H2B-tdTomato (white in colour). Arrowheads emphasize the movement of sperm cell nuclei just before and after pollen discharge and egg cell fertilization. Asterisk shows the timing of egg cell fertilization. Scale bar, 10 μm. Numbers indicate time (min) as in b . ( e ) Time course of the FRET/CFP ratio change shown in d . ( f ) Plot of the time difference between pollen tube discharge and first Ca 2+ peak ( n =28). ( g , h ) Plot of the timing of events relating the second Ca 2+ peak with EC fertilization ( g , n =24) or CC fertilization ( h , n =21). A regression line (dashed line) is shown. Full size image For imaging at higher temporal resolution, Förster resonance energy transfer (FRET)/cyan fluorescent protein (CFP) ratio imaging of ovules was performed at one to four frames per min using a spinning-disk confocal microscope equipped with automatic filter changer and high sensitive electron multiplying-charge coupled device (EM-CCD) camera ( Fig. 1d,e , Supplementary Fig. 1b ). Consistent with the observations made by two-photon excitation imaging, monitoring [Ca 2+ ]cyt of the egg cell in 15 s time-lapse intervals did not reveal an oscillatory pattern following fertilization as is typical for many animal gamete fusions, but instead two distinct, transient Ca 2+ spikes were observed ( Fig. 1d,e , Supplementary Movie 2 ). The data show that the first Ca 2+ peak corresponded to pollen tube discharge, whereas the second coincided with egg cell fertilization ( Fig. 1d,e ). No noticeable Ca 2+ elevation was detected in the egg cell at the time of central cell fertilization ( Fig. 1e ). The first peak in [Ca 2+ ]cyt was of relatively short duration (2.8±1.0 min) and occurred simultaneously in the entire egg cell without apparent starting location. The second peak seemed to start at the chalazal end where the fusion with the sperm cell occurs and then spread over the entire cell ( Fig. 1d ), consistent with observations made during in vitro fertilization of the maize eggs [10] . Remarkably, the duration of the second peak (4.7±1.2 min), while longer than the first, was much shorter than the peak observed in the in vitro fertilization system using maize (several tens of min to more than 1 h [10] , [20] ). Previously, we have shown that the order of egg cell and central cell fertilization is arbitrary [6] . Therefore, to substantiate the temporal correlation between individual events, we quantitatively analysed Ca 2+ dynamics in the egg cell using data from a total of 28 cases of pollen tube discharge, 24 cases of egg cell fertilization and 21 cases of central cell fertilization. The average time delay between pollen tube discharge and the first Ca 2+ peak was 2.3±15 s ( Fig. 1f ), clearly confirming that this first Ca 2+ peak corresponds to the timing of pollen tube discharge. The second Ca 2+ peak correlated much stronger with the moment of egg cell fertilization, which is indicated by a sudden movement of the sperm cell nucleus, than that of central cell fertilization ( Fig. 1g,h ) corroborating that this second Ca 2+ peak in the egg cell corresponds to the timing of its own fertilization. Distinct triggers of two Ca 2+ spikes in the egg cell The two spikes in [Ca 2+ ]cyt clearly seem to represent characteristic Ca 2+ dynamics of the egg cell during double fertilization. While the temporal correlation of these peaks with the events occurring in the male gametophyte was striking, we wanted to prove the existence of a causal relationship. To do so, we used a mutant of the GCS1/HAP2 gene, which encodes a highly conserved male gamete transmembrane protein in various eukaryotes including A. thaliana [21] , [22] . In the gcs1/hap2 −/+ mutant, pollen tube discharge occurs normally, but the sperm cells do not fuse with the egg or central cell, probably due to a defect in a step after the cell attachment [21] , [22] , [23] . In the semi- in vivo assay used here, the two sperm cells of the gcs1/hap2 mutant pollen do not indeed move towards or fuse with their targets but remain at the location where they were ejected ( Fig. 2a , Supplementary Movie 3 ). In these samples, only the first Ca 2+ spike was observed in the egg cell and no subsequent Ca 2+ spike was detected ( Fig. 2a,b ). In the absence of pollen tube discharge, no Ca 2+ spike was detected ( Supplementary Fig. 2a,b , Supplementary Movie 4 ). These observations are consistent with the first Ca 2+ peak being triggered by pollen tube discharge and the second peak requiring a gamete fusion event. 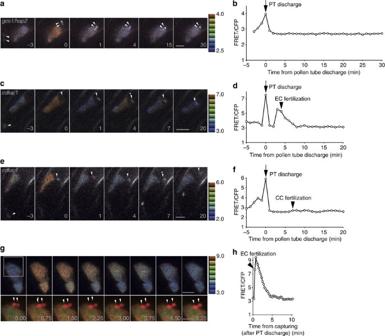Figure 2: The second Ca2+spike in the egg cell corresponds to egg cell fertilization. (a,c,e) Time-lapse series of confocal images (maximum projections of two or three optical sections) of the egg cell expressing YC3.60 receive sperm cells delivered fromgcs1/hap2(a) andcdka;1(c,e) mutant pollen tubes expressing pHTR10::HTR10-mRFP (white in colour). Representative FRET/CFP ratio images are shown as inFig. 1. Numbers indicate time (min) before and after the pollen tube discharge. Arrowheads indicate sperm cell nuclei. The single sperm cells in pollen tubes of thecdka;1mutant fertilized either egg cell (c) or central cell (e). Moment of fertilization is indicated by asterisk. Scale bar, 10 μm. (b,d,f) Time course of the FRET/CFP ratio change at the egg cell expressing YC3.60 shown in (a,c,e). (g) Time-lapse series of confocal optical sections of the egg cell expressing cytosol-associated YC3.60 and plasma membrane associated TagRFP-PIP2a and the sperm cell nucleus expressing pHTR10::HTR10-mRFP. Upper panel with representative FRET/CFP ratio images are shown as before. The square indicates the region shown in the lower panels. Lower panels show merged images of CFP (cyan), Venus (yellow) and mRFP (red). Arrowheads indicate sperm cell nuclei. Asterisk shows the timing of egg cell fertilization based on the timing of sperm cell nucleus movement across the plasma membrane of the egg cell. Representative FRET/CFP ratio images and numbers are shown as before. Scale bar, 10 μm. (h) Time course of the FRET/CFP ratio change at the egg cell expressing YC3.60 shown ing. Numbers indicate time (min) after the beginning of observation. Figure 2: The second Ca 2+ spike in the egg cell corresponds to egg cell fertilization. ( a , c , e ) Time-lapse series of confocal images (maximum projections of two or three optical sections) of the egg cell expressing YC3.60 receive sperm cells delivered from gcs1/hap2 ( a ) and cdka;1 ( c , e ) mutant pollen tubes expressing pHTR10::HTR10-mRFP (white in colour). Representative FRET/CFP ratio images are shown as in Fig. 1 . Numbers indicate time (min) before and after the pollen tube discharge. Arrowheads indicate sperm cell nuclei. The single sperm cells in pollen tubes of the cdka;1 mutant fertilized either egg cell ( c ) or central cell ( e ). Moment of fertilization is indicated by asterisk. Scale bar, 10 μm. ( b , d , f ) Time course of the FRET/CFP ratio change at the egg cell expressing YC3.60 shown in ( a , c , e ). ( g ) Time-lapse series of confocal optical sections of the egg cell expressing cytosol-associated YC3.60 and plasma membrane associated TagRFP-PIP2a and the sperm cell nucleus expressing pHTR10::HTR10-mRFP. Upper panel with representative FRET/CFP ratio images are shown as before. The square indicates the region shown in the lower panels. Lower panels show merged images of CFP (cyan), Venus (yellow) and mRFP (red). Arrowheads indicate sperm cell nuclei. Asterisk shows the timing of egg cell fertilization based on the timing of sperm cell nucleus movement across the plasma membrane of the egg cell. Representative FRET/CFP ratio images and numbers are shown as before. Scale bar, 10 μm. ( h ) Time course of the FRET/CFP ratio change at the egg cell expressing YC3.60 shown in g . Numbers indicate time (min) after the beginning of observation. Full size image On pollen tube discharge, both the pollen tube and the receptive synergid cell rupture, and their contents can be exposed to the egg cell [6] , [24] , which involves high concentration of Ca 2+ deriving from the synergid cell [24] , [25] . To examine whether such exposure to external Ca 2+ can trigger cytosolic Ca 2+ elevation in the egg cell, we performed laser disruption of one of the synergid cells in semi- in vivo cultivated ovules. The femtosecond pulse laser normally used for two-photon microscopy is able to disrupt a single cell within thick tissues by focusing high energy in short pulses without thermal damage [26] . Following such a laser-mediated disruption of a synergid cell, cytosolic Ca 2+ spikes in the egg cell were observed in eight cases out of 10 ( Supplementary Fig. 3a,b , Supplementary Movie 5 ). In contrast, when the central cell was disrupted in a similar fashion, only a weak Ca 2+ spike was observed in the egg ( n =6; Supplementary Fig. 3c,d , Supplementary Movie 6 ). To dissect the relationship between the second Ca 2+ spike and double fertilization, we next used an A-type cyclin-dependent kinase (cdka;1) mutant [27] , [28] . About 40% of the pollen tubes of the cdka;1 mutant only carry a single sperm cell [29] . This single sperm cell can fertilize either the egg cell (18.9%) or the central cell (5.8%) (ref. 29 ). In ovules in which the egg cell but not the central cell was fertilized by the cdka;1 single sperm cell, two Ca 2+ peaks were observed ( Fig. 2c,d , Supplementary Movie 7 ), with the timing of the second peak being correlated with the timing of the egg cell fertilization event ( Fig. 2d ). In contrast, when the central cell was fertilized by the cdka;1 single sperm cell, only one detectable Ca 2+ peak was observed and it temporally correlated with the moment of pollen tube discharge ( Fig. 2e,f , Supplementary Movie 8 ). These results clearly indicate that the second Ca 2+ peak in the egg cell depends on egg cell fertilization and is independent of central cell fertilization. To ascertain the relationship between the moment of gamete membrane fusion and the second Ca 2+ spike, a marker line labelling the egg cell plasma membrane by TagRFP [19] was combined with the cytosolic YC3.60 marker line. This enabled us to determine that the second Ca 2+ spike coincided with the movement of the sperm nucleus across the egg cell plasma membrane ( Fig. 2g,h , Supplementary Movie 9 ). This was consistent with the behaviour of the sperm cell nucleus and Ca 2+ elevation during in vitro fertilization in maize [7] , [10] . We conclude that the second Ca 2+ spike in the egg cell is associated with gametic fusion, that is, plasmogamy of the egg cell. Calcium spikes in the central cell To complement the data obtained in egg cells, we examined Ca 2+ dynamics in the other crucial cells of the female gametophyte, the central cell and the two synergid cells. Using cell-specific YC3.60 marker lines ( FWA promoter for the central cell and MYB98 promoter for the synergid cell) and spinning-disk confocal microscopy. In vitro fertilization assays performed in Nicotiana tabacum had not revealed any Ca 2+ peaks in the central cell [30] . When we observed the Ca 2+ levels in the central cell of Arabidopsis at 1 frame per min, we did not detect any Ca 2+ spikes (data not shown). However, image acquisition at two frames per min enabled us to detect Ca 2+ spikes under the experimental condition we used. Coinciding with the moment of pollen tube discharge, Ca 2+ spikes were observed in all samples ( n =13) ( Fig. 3a,b , Supplementary Movie 10 , Supplementary Fig. 1c ). After pollen tube discharge, a second Ca 2+ spike was observed in 10 of 19 samples ( Supplementary Table 1 ). The duration of the second spike was 1.7±0.7 min and as in the case of the egg cell, no oscillatory pattern was observed following fertilization in the central cell. Occasionally, the second peak correlated with central fertilization (4 of 10) but in others it coincided with egg cell fertilization (5 of 10 including two cases of simultaneous double fertilization; Supplementary Table 1 ). In two of 10 cases, second peaks correlated with neither egg cell fertilization nor central cell fertilization. However, we never observed a Ca 2+ spike in the central cell before pollen tube discharge ( n =8 which observed at least 20 min before pollen tube discharge). 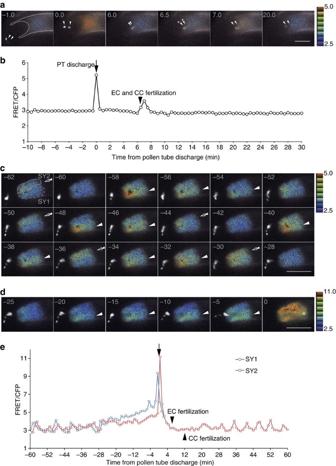Figure 3: The central cell shows similar Ca2+spike pattern as the egg cell, but the synergid cells show unique Ca2+oscillations. (a) Time-lapse series of confocal images (maximum projections of two optical sections) of the central cell expressing pFWA::YC3.60 fertilized by sperm cell nuclei labelled with pHTR10::HTR10-mRFP (white in colour). Representative FRET/CFP ratio images are shown as before. Arrowheads indicate the sperm cell nuclei. Asterisk shows the timing of egg cell and central cell fertilization, respectively. Numbers indicate time (min) as inFig. 1. Scale bar, 20 μm. (b) Time course of the FRET/CFP ratio change in the central cell expressing YC3.60 shown ina. In this case, egg cell fertilization and central cell fertilization occurred simultaneously. (c) Time-lapse series of confocal images (maximum projections of four optical sections) of the synergid cells expressing pMYB98::YC3.60 shows alternative Ca2+oscillations after pollen tube contact. Sperm cell nuclei were labelled with pRPS5A::H2B-tdTomato (white in colour). Representative FRET/CFP ratio images are shown as before. Arrowheads indicate Ca2+elevation in the synergid cell 1 and double arrowheads show that of the synergid cell 2. Numbers indicate time (min) as inFig. 1. Scale bar, 20 μm. (d) Just before the pollen tube discharge, Ca2+level in the synergid cell 1 (receiving pollen tube) increases more (emphasized in arrowheads) than that of synergid cell 2 (persistent after pollen tube discharge). Numbers indicate time (min) as inFig. 1. Scale bar, 20 μm. (e) Time course of the FRET/CFP ratio change in the two synergid cells expressing YC3.60 shown in (c,d). SY1 identifies the degenerated synergid cell and SY2 indicates the synergid cell that persists after pollen tube discharge. Figure 3: The central cell shows similar Ca 2+ spike pattern as the egg cell, but the synergid cells show unique Ca 2+ oscillations. ( a ) Time-lapse series of confocal images (maximum projections of two optical sections) of the central cell expressing pFWA::YC3.60 fertilized by sperm cell nuclei labelled with pHTR10::HTR10-mRFP (white in colour). Representative FRET/CFP ratio images are shown as before. Arrowheads indicate the sperm cell nuclei. Asterisk shows the timing of egg cell and central cell fertilization, respectively. Numbers indicate time (min) as in Fig. 1 . Scale bar, 20 μm. ( b ) Time course of the FRET/CFP ratio change in the central cell expressing YC3.60 shown in a . In this case, egg cell fertilization and central cell fertilization occurred simultaneously. ( c ) Time-lapse series of confocal images (maximum projections of four optical sections) of the synergid cells expressing pMYB98::YC3.60 shows alternative Ca 2+ oscillations after pollen tube contact. Sperm cell nuclei were labelled with pRPS5A::H2B-tdTomato (white in colour). Representative FRET/CFP ratio images are shown as before. Arrowheads indicate Ca 2+ elevation in the synergid cell 1 and double arrowheads show that of the synergid cell 2. Numbers indicate time (min) as in Fig. 1 . Scale bar, 20 μm. ( d ) Just before the pollen tube discharge, Ca 2+ level in the synergid cell 1 (receiving pollen tube) increases more (emphasized in arrowheads) than that of synergid cell 2 (persistent after pollen tube discharge). Numbers indicate time (min) as in Fig. 1 . Scale bar, 20 μm. ( e ) Time course of the FRET/CFP ratio change in the two synergid cells expressing YC3.60 shown in ( c , d ). SY1 identifies the degenerated synergid cell and SY2 indicates the synergid cell that persists after pollen tube discharge. Full size image Distinct calcium oscillations in the two synergid cells It was suggested that Ca 2+ oscillation and burst occur in the synergid cell at pollen tube arrival and discharge, respectively [14] , but the two synergid cells were not studied individually. In our setup, we were able to simultaneously monitor Ca 2+ dynamics in the two synergid cells in those 18 samples where these could be distinguished ( Fig. 3c,d , Supplementary Fig. 3d,e ). Before pollen tube arrival at the ovule, no oscillatory signal was detected under the experimental condition we used ( n =3), consistent with the previous report [14] . When a pollen tube contacted the synergid cell, alternating Ca 2+ oscillations occurred in the two synergid cells with the FRET/CFP ratio being similar in the two cells ( Fig. 3c,e , Supplementary Movie 11 ). Just before pollen tube discharge, Ca 2+ oscillation stopped and continuous, rapid elevation of cytosolic Ca 2+ occurred in both synergid cells. Interestingly, the Ca 2+ level in the receptive synergid cell before pollen tube discharge was higher than in the persistent synergid cell in 12 of 18 samples, suggesting that the receptive synergid is predetermined before pollen tube discharge. Immediately following pollen tube discharge, both synergids displayed sharp, short lived Ca 2+ peaks followed by a rapid return to the earlier Ca 2+ levels. To our surprise, the persistent synergid cell started oscillation again after double fertilization occurred ( Fig. 3e , Supplementary Movie 11 , Supplementary Fig. 4 ). We observed Ca 2+ dynamics in all the female gametophytic cells directly involved in the double fertilization of Arabidopsis . The egg cell displayed two distinct spikes on pollen tube discharge and gamete fusion, respectively. To examine the origin of the first Ca 2+ spike, we performed cell disruption analysis. When one of the two synergid cells was disrupted using laser, a transient Ca 2+ spike was detected in the egg cell, but no distinct signal was detected when the central cell was disrupted. It has been reported that synergid cells contain a high concentration of Ca 2+ in their cytosol compared with the other female gametophyte cells [24] , [31] . Disruption of the synergid cell might therefore have caused an elevation of the external Ca 2+ that was sufficient to cause the cytosolic Ca 2+ concentration in the egg to spike. On the other hand, it has been reported that mechanical stimulation can trigger cytosolic Ca 2+ elevation [32] . When one of the two synergid cells was disrupted, it immediately shrank ( Supplementary Movie 5 ), a phenomenon that resembles that of pollen tube discharge. Therefore, another possibility is that the mechanical stimulation resulting from synergid cell disruption might have caused cytosolic Ca 2+ elevation in the egg cell. Taken together, our data suggest that the first Ca 2+ spike in the egg cell is at least partly due to synergid cell degeneration triggered by pollen tube discharge and is independent of fertilization. High cytosolic concentration of Ca 2+ at the tip of the pollen tube [14] and mechanical pressure by the discharged pollen tube contents [6] are also possibly involved in the Ca 2+ spike of the egg cell during pollen tube discharge. The egg cell is known to secrete an EC1 peptide following pollen tube discharge but before fertilization. This peptide has been reported to activate sperm cells for fusion [33] . It is therefore reasonable to speculate that the egg cell senses pollen tube discharge and this Ca 2+ spike triggers peptide secretion. In animals like frogs and several marine invertebrates, polyspermy (the fertilization of an egg by two or more sperm cells) is prevented by an electrical charge across the surface of the egg (fast block in a few seconds) and/or by modification of the extracellular egg coat by a secretion reaction (slow block in dozens of seconds), following gamete fusion [34] . A Ca 2+ wave in the fertilized egg triggers the secretion reaction associated with the slow polyspermy block [34] . In the flowering plants, the mechanism of polyspermy block is unknown. However, the phenomenon was recognized by in vitro fertilization analysis in maize about 20 years ago [7] . Recent genetic approaches suggest the existence of a polyspermy block for both female gametes with the block in the egg cell being stronger than that in the central cell [13] . We speculate that the second Ca 2+ spike during fertilization of A. thaliana might be involved in blocking polyspermy. The fact that the Ca 2+ peak was observed simultaneously with the movement of the sperm nucleus across the plasma membrane of the egg cell at an image acquisition rate of four frames per min ( Fig. 2g,h ), suggests that Ca 2+ elevation begins within seconds after gamete fusion. The origin of this cytosolic Ca 2+ peak remains elusive. However, in the maize in vitro system using isolated egg cells, the origin of the [Ca 2+ ]cyt elevation in the fertilized egg cell has been suggested to be an intracellular Ca 2+ store rather than global influx from the outside [20] . Interestingly, the first Ca 2+ spike on pollen tube discharge does not seem to be involved in blocking polyspermy because discharge by gcs1/hap2 pollen tubes does not inhibit fertilization by a second, wild-type pollen tube even when its arrival and discharge occur several hours later [35] . Hence, the two Ca 2+ peaks, triggered by pollen tube discharge and fertilization, respectively, seem to have different physiological roles. Unlike most animal eggs, no oscillations of Ca 2+ were observed in the fertilized egg cell of A. thaliana. After the single fertilization-induced Ca 2+ peak, [Ca 2+ ]cyt decreased to a resting level within 4.7±1.2 min and no subsequent peak was observed for at least 45 min after fertilization. It cannot be excluded that there might be other spikes that could not be detected in our 15–30 s time-lapse in vivo imaging, but no oscillation was detected in the in vitro system using isolated maize eggs either [10] , [20] nor in independent work on the Arabidopsis female gametophyte using a different Ca 2+ probe [36] . This is consistent with previous in vitro fertilization analyses that showed no subsequent peak for at least 50 min after fertilization [10] . The presence of a single pulse of Ca 2+ rather than oscillations during gamete fusion has been reported in some animal species, for example cnidarians, echinoderms, fish and frogs [3] . However, in these species, a single Ca 2+ pulse typically fails to fully activate the oocytes, whereas multiple Ca 2+ spikes tend to successfully release oocytes from meiotic arrest to form both polar bodies [37] , [38] , [39] . Multiple spikes are likely to provide a more robust trigger, and the pattern of Ca 2+ spikes might depend on the necessity of a resumption from meiotic arrest [3] . In flowering plants, no resumption from meiotic arrest is required [40] . Instead, flowering plants show unique cell cycle control in fertilization among eukaryotes; sperm cells of Arabidopsis in G2 phase have been proposed to fuse with the egg cell in G1/S or G2 phase and with the central cell in G2 phase [41] . Different mechanisms of cell cycle arrest and activation might exist. Moreover, the transcriptional activation of male and female genomes in the zygote is critical for establishing apical–basal cell polarity over a long period of time before the first division [42] , [43] . Our data suggest that unlike egg cell functioning in animals such as hamster, in Arabidopsis , a single spike of [Ca 2+ ]cyt at fertilization with a duration that is much shorter than that observed during maize in vitro fertilization [7] , [20] , might be sufficient for blocking polyspermy and initiation of the developmental programme. The other female gamete, the central cell, showed a Ca 2+ peak correlated with pollen tube discharge and sometimes showed a second Ca 2+ spike, which did not display any consistent correlation with the timing of the central cell fertilization or that of egg cell fertilization. It can be stated, however, that the second Ca 2+ spike in the central cell is related to the gametic phase of double fertilization after the release of the sperm cells. Determination of fertilization targets during the gametic phase of double fertilization is still largely unknown but must require complex gamete recognition and/or blocking polyspermy in both female gametes [13] . The second Ca 2+ spike observed in the central cell might reveal unidentified cell-to-cell communication in double fertilization, although development of a high-speed and high-sensitivity microscope system will be necessary to detect faint Ca 2+ spikes efficiently. Both synergid cells showed Ca 2+ oscillation after pollen tube arrival, but before pollen tube discharge, with the receptive synergid cell showing superior Ca 2+ elevation (flooding) confirming independent studies [36] , [44] . Components of the FERONIA receptor kinase signalling pathway are required for appropriate calcium dynamics in the synergid cells [44] . The Ca 2+ elevation in the receptive synergid cell might be involved not only in its subsequent degeneration [5] but also in the interaction with the pollen tube by extruding Ca 2+ through calcium channels, which in turn trigger pollen tube rupture [45] . On pollen tube discharge, a strong Ca 2+ spike was observed in both synergid cells. This Ca 2+ spike might result from the breakdown of the receptive synergid cell including its vacuole and/or from the mechanical stimulation during pollen tube discharge [24] . To our surprise, an onset of Ca 2+ oscillation in the persistent synergid cell following double fertilization was observed. Completion of fertilization in the two female gametes independently, but additively, suppresses the attraction activity of the persistent synergid cell [46] , which eventually degenerates during the onset of seed development [47] . It is conceivable that Ca 2+ oscillation in the persistent synergid cell is triggered by fertilization of the female gametes and that this Ca 2+ signature is involved in the cessation of synergid cell function. To summarize, we revealed distinct Ca 2+ dynamics in the crucial female gametophytic cells during double fertilization. In the future, new technology such as optical manipulation of Ca 2+ spiking [48] may provide insights into physiological roles of the Ca 2+ signalling observed in this study. Knowledge of these Ca 2+ dynamics and their physiological roles will accelerate the identification of key molecules involved in intra- and intercellular signalling during double fertilization. Plant materials and growth conditions A. thaliana ecotype Columbia (Col-0) was used as the wild type. The pHTR10::HTR10-mRFP [6] , pRPS5A::H2B-tdTomato [49] , pDD45::TagRFP-PIP2a [19] , gcs1/hap2 −/+ (ref. 21 ) and cdka;1 −/+ (ref. 27 ) lines have been described previously. Seeds were sterilized with 5% sodium hypochlorite containing 0.5% Triton X-100 and germinated on plates containing 0.5 × Murashige and Skoog salt (pH 5.7; Wako Pure Chemical, Osaka, Japan), 2% sucrose, Gamborg’s B5 vitamin solution (Sigma) and 0.3% Gerlite (Wako Pure Chemical) in a growth chamber at 22 °C under 24-h light after cold treatment (4 °C) for 2 days. Ten-day-old seedlings were transferred to soil (Hanachan-baiyoudo; HANAGOKORO, Nagoya, Japan) and grown at 22 °C under 24-h light. Semi -in vivo fertilization assay Pollen tube growth medium (14% sucrose, 0.001% boric acid, 1.27 mM Ca(NO 3 ) 2 , 0.4 mM MgSO 4 , 1.5% agarose (50081; Lonza) and adjusted to pH 7.0 with KOH) was used for the semi -in vivo fertilization assay. For the well, 1-mm thick silicon rubber (6-611-02, AsOne) was placed on a 2,550-mm coverslip (C025501, Matsunami). About 150 μl of medium melted at 65 °C was poured into the well, and covered with another coverslip. Flowers were emasculated 12–18 h before hand pollination. Pistils held on a glass slide with double-sided tape were hand pollinated under a stereomicroscope, and cut with a 27-gauge needle (NN-2738R, Terumo) at the junction between the style and ovary, and placed on the medium. The pistils were excised ovules with a 0.5-mm-diameter insect pin. The ovules were placed immediately on the medium within 2 mm of the distance from the pistil. Double fertilization was observed 5–8 h after pollination at 20 °C in the dark. Vector construction The YC3.60 coding sequence followed by the nopaline synthase terminator (NosT) was digested with Bam HI and Eco RI from pACT1::YC3.60 vector [50] and cloned into the binary vector pPZP211 (ref. 51 ) using Bam HI and Eco RI sites, resulting in pPZP211-YC3.60. The YC3.60 coding sequence was also digested with Bam HI and Sac I from pACT1::YC3.60 vector and cloned into a subcloning vector pBlueMAP [42] derivative in which multiple cloning sites located between Asc I sites were replaced by multiple cloning sites from the pPZP vector followed by NosT sequence, resulting in pBlueMAP-YC3.60. Promoter regions of MYB98 (ref. 52 ), FWA [53] and DD45 (ref. 16 ) were amplified by PCR from genomic DNA with primer pairs (5′- caccaagcttGGTGAAGAGAGAGAGAGAGA -3′ and 5′- cgcggatccGTGTTCTTGATCACGTGTGAAG -3′ for MYB98 promoter; 5′- cccaagcttGGTAGGCTAATAATCAGAAGCCC -3′ and 5′- cgggatccTTTCCCTCAATGCAATAACCTG -3′ for FWA promoter; 5′- ggagtcgacCTCAGAGAACATGAACGGGTC -3′ and 5′- ggagtcgacTATTCTTTCTTTTTGGGGTTTTTG -3′ for DD45 promoter). The MYB98 and FWA promoters were inserted into the pPZP211-YC3.60 using Hin dIII and Bam HI, resulting in the binary vectors pPZP211-pMYB98::YC3.60 and pPZP211-pFWA::YC3.60. The DD45 promoter was subcloned in the pBlueMAP-YC3.60 using Sal I. A cassette containing the DD45 promoter followed by YC3.60 and NosT was cut with Asc I and ligated in a pMDC99 (ref. 54 ) derivative in which ccdB was removed by Eco RI digestion and self-ligation, resulting in the binary vector pMDC99-pDD45::YC3.60. The binary vectors pPZP211-pMYB98::YC3.60, pPZP211-pFWA::YC3.60 and pMDC99-pDD45::YC3.60 were introduced into Agrobacterium tumefaciens strain GV3101 and then transformed into wild-type A. thaliana plants (Col-0) using the floral dip method. Transformed plants were selected on Murashige-Skoog plates containing 50 μg per 1 ml kanamycin for pPZP211-pMYB98::YC3.60 and pPZP211-pFWA::YC3.60 or 20 μg per 1 ml hygromycin B for pMDC99-pDD45::YC3.60. Microscopy settings For calcium imaging, we used four microscope systems: spinning-disk confocal microscopes, laser scanning confocal microscope and two-photon excitation microscope. Confocal images were acquired using an inverted microscope (IX-81; Olympus, Tokyo, Japan) equipped with an automatically programmable XY stage (MD-XY30100T-Meta; Molecular Devices, Sunnyvale, CA), a spinning-disk confocal system (CSU-X1; Yokogawa Electric, Tokyo, Japan), 445 nm (Stradus; Vortran Laser Technologies, Sacramento, CA) and 561 nm (Sapphire; Coherent, Santa Clara, CA) LD lasers and EM-CCD camera (Evolve 512, Photometrics, Tucson, AZ). Time-lapse images were acquired every 10–60 s using multiple z-planes (3.0-μm intervals) and three to 11 planes with a × 40 water-immersion objective lens (UApo 40XW3/340, WD=0.25 mm, NA=1.15; Olympus) or with a × 60 silicone immersion objective lens (UPLSAPO60XS, WD=0.30 mm, NA=1.30; Olympus) mounted on a Piezo focus drive (P-721; Physik Instrumente, Karlsruhe, Germany). For rapid imaging, the images were acquired every 10–15 s with single z plane. Exposure times were 100–300 ms for CFP and Venus, and 50–100 ms for mRFP. We used three band-pass filters, 482/35 nm for CFP, 578/105 nm for Venus and 600/37 nm for mRFP. Images were processed with Metamorph (Universal Imaging Corp., Downingtown, PA) to create maximum intensity projection images and to add colour. For split-view imaging, we used an inverted microscope (IX-81; Olympus) equipped with an automatically programmable XY stage (BioPrecision; Ludl Electronic Products Ltd, Hawthorne, NY), a spinning-disk confocal system (CSU-W1; Yokogawa Electric), 445 nm (Stradus; Vortran Laser Technologies) and 561 nm (Sapphire; Coherent) LD lasers and EM-CCD camera (ImagEM 1K; Hamamatsu Photonics, Shizuoka, Japan). Time-lapse images were acquired every 10–60 s using multiple z-planes (3.0-μm intervals) and three to 11 planes with a × 40 water-immersion objective lens (UApo 40XW3/340) or with a × 60 silicone immersion objective lens (UPLSAPO60XS). For rapid imaging, the images were acquired every 10–15 s with single z plane. Exposure times were 100–300 ms for CFP and Venus, and 50–100 ms for mRFP. We used three band-pass filters, 482/35 nm for CFP, 578/105 nm for Venus and 600/37 nm for mRFP. Images were processed with Metamorph (Universal Imaging Corp.) to create maximum intensity projection images and to add colour. For laser disruption, we used a laser scanning inverted microscope (LSM780-DUO-NLO; Zeiss, Göttingen, Germany) equipped with a Ti-Sapphire femtosecond pulse laser (Chameleon Vision II; Coherent). A Ti:sapphire laser tuned to 800 nm was used for disruption and excitation. To disrupt single cells, the targets were irradiated by femtosecond pulse laser with one-frame scanning. Before and after laser irradiation, time-lapse images were acquired using single z plane with a × 40 water-immersion objective lens (LD C-APOCHROMAT, WD=0.62 mm, NA=1.10; Zeiss). The images were acquired every 15 s at 250 ms per scan. Each image is the average of two lines. Emitted fluorescence signals were detected by the external Non-Descanned GaAsP Detectors. We used a filterset for CFP/YFP (1756-084; Zeiss), 460–500 nm for CFP, 525–560 nm for Venus. The images were acquired and analysed using the ZEN 2010 software (Zeiss). Two-photon images were acquired using a laser scanning inverted microscope (A1R MP; Nikon, Tokyo, Japan) equipped with a Ti-Sapphire femtosecond pulse laser (Mai Tai DeepSee; Spectra-Physics, Mountain View, CA). A Ti:sapphire laser tuned to 800 nm was used for excitation. Time-lapse images were acquired using multiple z -planes (2.0 or 3.0 μm intervals) and four to eight planes with a × 40 water-immersion objective lens (CFI Apo LWD × 40 WI, WD=0.61 mm, NA=1.15; Nikon). The images were acquired every 60 s at 500 ms per scan. Each image is the average of two lines. Emitted fluorescence signals were detected by the external Non-Descanned PMT Detectors. We used two dichroic mirrors, DM495 and DM560, and three band-pass filters, 479/40 nm for CFP, 534/30 nm for Venus, and 578/105 nm for mRFP. The images were acquired and analysed using the NIS-Elements AR software 4.10 (Nikon). Image processing All images were adjusted for brightness and contrast by Adobe Photoshop CS4 (Adobe Systems, Inc., San Jose, CA). MacBiophotonics ImageJ software ( http://www.macbiophotonics.ca/ ) was used for editing of the images and movies. Images were aligned to correct for experimental drift using the ImageJ plugin ‘align slices in stack’ ( https://sites.google.com/site/qingzongtseng/template-matching-ij-plugin ). For FRET pixel-to-pixel ratiometric processing and efficiency analysis, corrected FRET images were obtained by using the FRET dialogue feature of Metamorph (Universal Imaging Corp.). CFP and FRET emissions were summed over an entire cell after background subtraction, and the FRET:CFP emission ratio was calculated. Representative FRET/CFP ratio images are shown in the intensity modulated display mode with 32-intensity in 8-ratio. How to cite this article: Hamamura, Y. et al . Live imaging of calcium spikes during double fertilization in Arabidopsis . Nat. Commun. 5:4722 doi: 10.1038/ncomms5722 (2014).